Wittichenite semiconductor of Cu3BiS3films for efficient hydrogen evolution from solar driven photoelectrochemical water splitting A highly efficient, low-cost and environmentally friendly photocathode with long-term stability is the goal of practical solar hydrogen evolution applications. Here, we found that the Cu 3 BiS 3 film-based photocathode meets the abovementioned requirements. The Cu 3 BiS 3 -based photocathode presents a remarkable onset potential over 0.9 V RHE with excellent photoelectrochemical current densities (~7 mA/cm 2 under 0 V RHE ) and appreciable 10-hour long-term stability in neutral water solutions. This high onset potential of the Cu 3 BiS 3 -based photocathode directly results in a good unbiased operating photocurrent of ~1.6 mA/cm 2 assisted by the BiVO 4 photoanode. A tandem device of Cu 3 BiS 3 -BiVO 4 with an unbiased solar-to-hydrogen conversion efficiency of 2.04% is presented. This tandem device also presents high stability over 20 hours. Ultimately, a 5 × 5 cm 2 large Cu 3 BiS 3 -BiVO 4 tandem device module is fabricated for standalone overall solar water splitting with a long-term stability of 60 hours. Solar water splitting using sunlight irradiation has been widely believed to be a clean way to produce hydrogen energy without CO 2 emission [1] , [2] , [3] , [4] . As an appreciable solar energy utilization/conversion mode, photoelectrochemical (PEC) solar water splitting has been extensively studied based on various semiconductors [5] , [6] , [7] . Since Honda and Fujishima found that TiO 2 photoelectrodes showed promising PEC water splitting properties [8] , various semiconductor materials have been investigated to improve the solar-to-hydrogen (STH) conversion efficiency and device working stability [9] . The core of the PEC water splitting device is at the semiconductor/liquid interface junction, where minority carriers excited in the semiconductor are driven into the liquid by the electric field in the depletion region at the semiconductor/liquid interface [6] . For example, redox reactions, such as the reduction of H + to H 2 , are driven at the interface between the P-type semiconductor and liquid. To date, many p-type semiconductors have been studied as photocathodes for PEC water splitting. P-type semiconductors that are used on photovoltaic devices such as c-Si [10] , a-Si [11] , Cu(In,Ga)Se [12] , [13] , CuInS 2 [14] , Cu 2 ZnSnS 4 (CZTS) [15] , [16] , CuSbS 2 [17] , Sb 2 Se 3 [18] and CdTe [19] are always suitable as the photocathode for PEC water splitting due to their high light absorption coefficient and suitable optical band gap. In recent years, Cu-chalcogenide compound semiconductors have attracted wide attention for PEC water splitting. Although Cu-chalcogenide photocathodes such as CuInS 2 [14] , CuGaSe 2 [20] , CuGa 3 Se 5 [21] , (Ag,Cu)GaSe 2 [22] , and Cu(In,Ga)Se 2 [12] , [13] , show excellent STH conversion efficiency, there are many difficulties in their large-scale production with regards to low throughput and material utilization because of the limited availability of elements (i.e., In, Ga and Se). Therefore, cost-effective and environmentally protective CZTS semiconductors are believed to be promising photocathode materials that have been investigated for ~10 years since the first report from Prof. Domen’s group in 2010 [23] . During the last few years, many researchers, including us, have made efforts to improve the STH conversion efficiency and working stability [15] , [16] , [24] , [25] , [26] , [27] , [28] . Recently, we achieved a record applied bias photon-to-current efficiency (ABPE) over 2.7% and 3.5% with the highest onset potential of 0.7 V RHE and over 10 h of PEC stability for the CZTS-based photocathode by various surface modifications [25] , [28] . However, the complex element consistency and numerous antisite/vacancy defects of CZTS compounds restrict their photovoltage. The record onset potential we achieved at ~0.7 V RHE is still not appreciable for the further fabrication of efficient tandem cells with suitable photoanodes such as BiVO 4 and Fe 2 O 3 [29] , [30] . Meanwhile, the required postsulfurization process of the CZTS film also restricted its large-scale industrial integration for solar hydrogen evolution [16] , [25] , [28] . Cu 2 O-based photocathodes have been widely investigated due to their high PEC photovoltage, which has reached as high as 1.2 V RHE , but their low stability is still a major problem [31] , [32] . Fortunately, ternary I − V − VI compounds of Cu 3 BiS 3 are believed to be promising chalcogenide compounds for photovoltaic devices due to their perfect optical band gap ( Eg ≈ 1.4–1.7 eV), high absorption coefficient (>10 5 cm −1 ) compared to those of CuInSe 2 and Cu 2 ZnSnS 4 , and p-type conductivity with a carrier concentration of ~2 × 10 16 cm −3 [33] , [34] , [35] . Cu 3 BiS 3 , naturally occurring in the “Wittichenite” mineral form, is stable for a broad range of processing temperatures [36] . Moreover, it is made of inexpensive, nontoxic, and earth-abundant elements, and we found that the Cu 3 BiS 3 film can be easily produced on a large scale by any suitable low-cost approach not under vacuum, such as printing and spraying [34] , [37] . Recently, Cu 3 BiS 3 has attracted much attention, and remarkable progress has been made by many groups using different fabrication approaches and theoretical studies [38] , [39] , [40] . However, the previously reported photovoltaic performances and PEC water splitting efficiencies of Cu 3 BiS 3 -based solar cells or photocathode devices are still not significant [35] , [37] , [38] , [39] . The best conversion efficiency achieved by a Cu 3 BiS 3 -based solar cell is 0.17% (0.11 cm 2 active area) [37] , and the best reported Cu 3 BiS 3 -based photocathode only presented a 0.1 mA/cm 2 photocurrent density at 0 V RHE ( J 0 ), with a 0.65 V RHE onset potential value ( Voc ) [38] . Moreover, the reported devices are all on the lab scale, and their stabilities are all not appreciable (<60 min) [37] , [38] , [39] . The reported low efficiency and poor PEC performance of Cu 3 BiS 3 -based photoelectrodes are far from their theoretical limit considering their perfect optical band gap value of ~1.7 eV for solar water splitting, and the low working stability itself restricts their further industrial utilization [38] , [39] . The low solar-to -hydrogen conversion efficiency should be caused by the low crystallinity of the material, poor surface/interface conditions and obvious internal defects [33] , [38] . In this work, we presented a world record ABPE of 1.7% for our Cu 3 BiS 3 -based photocathode for solar water splitting, and the photocurrent density ( J 0 ) of ~7 mA/cm 2 , onset potential ( Voc ) of 0.9 V RHE and ABPE of 1.7%. The obtained photocurrent density ( J 0 ) of ~7 mA/cm 2 are almost 70 times higher than their previously reported highest values of J 0 (0.1 mA/cm 2 ) [38] . In addition, due to the high onset potential of the Cu 3 BiS 3 -based photocathode, we first fabricated a tandem cell of Cu 3 BiS 3 -BiVO 4 for unbiased solar water splitting, and an unassisted bright STH conversion efficiency over 2% was also achieved. More importantly, a large-scale Cu 3 BiS 3 -based single photocathode over 5 × 5 cm 2 was also fabricated. Finally, with the help of the BiVO 4 photoanode, a large 5 × 5 cm 2 Cu 3 BiS 3 -BiVO 4 tandem cell was fabricated. We were excited to find that the large-scale Cu 3 BiS 3 -BiVO 4 tandem cell showed long-term working stability, and the device working stability was found to be very high; the solar water splitting photocurrents were not degraded over 60 h (70% of their initial photocurrent density was maintained). This is the first report of an efficient and large-sized Cu 3 BiS 3 -based photocathode and Cu 3 BiS 3 -BiVO 4 tandem cell for unbiased solar water splitting. The large device size, appreciable STH conversion efficiency and high device working stability that were presented in this work indicated the promising practical application potentials of the Cu 3 BiS 3 -based photoelectrode. Fabrication and optimization of the Cu 3 BiS 3 thin films In this work, Cu 3 BiS 3 thin films were prepared by spray pyrolysis in one step. The detailed raw materials and process for the preparation of Cu 3 BiS 3 films are given in the Supporting Information . We found that the quality of the Cu 3 BiS 3 films was significantly influenced by the substrate temperature and Cu: Bi molar ratio of the precursor solution. 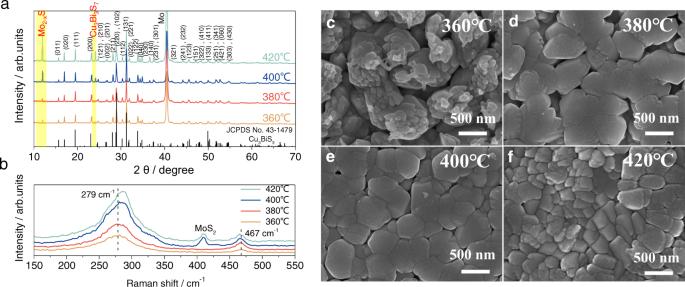Fig. 1: Structural characterization of the Cu3BiS3thin films. (a) XRD patterns and (b) Raman spectra of the Cu3BiS3films sprayed at various substrate temperatures. surface SEM images of the Cu3BiS3films sprayed at various substrate temperatures of (c) 360 °C, (d) 380 °C, (e) 400 °C and (f) 420 °C. Source data are provided as aSource Data file. Figure 1a shows the XRD patterns of the Cu 3 BiS 3 films sprayed at various substrate temperatures (360 °C, 380 °C, 400 °C and 420 °C). It was found that the intensity of major diffraction peaks increased with increasing substrate temperature, indicating that the crystallinity of Cu 3 BiS 3 films was improved with the substrate temperature. Nevertheless, some impurity phases, such as Mo 2-x S and Cu 3 Bi 3 S 7, were also easily formed at high substrate temperatures (marked with a yellow background in Fig. 1a ). Furthermore, the substrate temperature-dependent Raman spectrum of the Cu 3 BiS 3 films is shown in Fig. 1b . We observed two major vibrational peaks at 279 cm −1 and 467 cm −1 from the Raman spectrum, which matched well with the reported Raman shifts of Cu 3 BiS 3 films [33] , [38] . The half-widths of the vibrational peaks at ~279 cm −1 and 467 cm −1 decreased with increasing substrate temperature, indicating that the crystallinity increased with increasing substrate temperature. In addition, an extra Raman shift peak at ~410 cm −1 (corresponding to the MoS 2 Raman peak) appeared when the substrate temperature increased to above 400 °C. Notably, post-high-temperature sulfurization is generally necessary for the further crystal growth of multimetal sulfide materials [13] , [14] , [15] , [16] , [17] . Nevertheless, the one-step sprayed Cu 3 BiS 3 films in this work possessed good crystalline quality and pure phases with no obvious secondary phase or impurity phase, indicating that no postannealing process was required, which was instrumental in scalability and practical applications for Cu 3 BiS 3 -based photocathodes. Fig. 1: Structural characterization of the Cu 3 BiS 3 thin films. ( a ) XRD patterns and ( b ) Raman spectra of the Cu 3 BiS 3 films sprayed at various substrate temperatures. surface SEM images of the Cu 3 BiS 3 films sprayed at various substrate temperatures of ( c ) 360 °C, ( d ) 380 °C, ( e ) 400 °C and ( f ) 420 °C. Source data are provided as a Source Data file . Full size image The microstructural morphologies of the Cu 3 BiS 3 films sprayed at various substrate temperatures (360 °C, 380 °C, 400 °C and 420 °C) are shown in Fig. 1c–f . The films sprayed at a relatively low substrate temperature of 360 °C were not compact, various small crystals composed the Cu 3 BiS 3 films, and obvious fluctuations with large gaps were observed from their surface morphology (Fig. 1c ). When we increased the substrate temperature to 380 °C, the Cu 3 BiS 3 crystal size significantly increased to ~1000 nm, and the films were observed to be compact and flat (Fig. 1d ). Although the Cu 3 BiS 3 films sprayed at 400 °C were dense and smooth, the crystal size of Cu 3 BiS 3 was slightly decreased (Fig. 1e ). Moreover, when the substrate temperature increased to 420 °C, the size of the Cu 3 BiS 3 crystals obviously decreased to ~300–500 nm (Fig. 1f ). 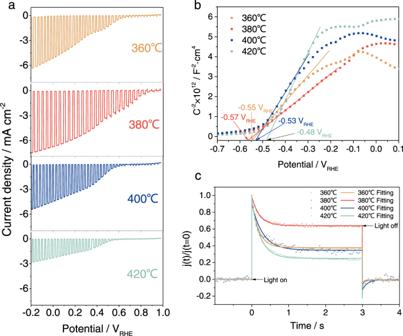Fig. 2: Performance and charge transfer dynamics characterization of the Cu3BiS3-based photocathode sprayed at various substrate temperatures. (a) Chopped photocurrent density-potential curves, (b) corresponding Mott–Schottky curves and (c) corresponding transit photocurrent spectra of the Cu3BiS3-based photocathodes sprayed at various substrate temperatures (360 °C, 380 °C, 400 °C and 420 °C). Source data are provided as aSource Data file. Figure 2a shows the PEC performance of the Cu 3 BiS 3 -based photocathodes sprayed at various substrate temperatures determined by LSV under chopped sunlight irradiation. The photocathode based on the Cu 3 BiS 3 film sprayed at 380 °C exhibited the highest photocurrent density (~7 mA/cm 2 ), onset potential (~0.9 V RHE ) and fill factor. Meanwhile, the statistical plots shown in Fig. S1 also persuasively suggested this trend. The flat band potential ( V fb ) of the Cu 3 BiS 3 -based photocathodes sprayed at various substrate temperatures can be determined from the intersecting points of the Mott–Schottky curves and X axis (shown in Fig. 2b ) [41] . The photocathodes based on the Cu 3 BiS 3 films sprayed at 360 °C, 380 °C, 400 °C and 420 °C exhibited V fb values of −0.55 V RHE , −0.57 V RHE , −0.53 V RHE and −0.48 V RHE , respectively. The most negative Vfb of −0.57 V RHE (corresponding to the photocathode based on the Cu 3 BiS 3 film sprayed at 380 °C) implied the highest energy level of photogenerated electrons, indicating that it was easier for photogenerated electrons to transfer from the electrode into the electrolyte and participate in the hydrogen evolution reaction [41] . Fig. 2: Performance and charge transfer dynamics characterization of the Cu 3 BiS 3 -based photocathode sprayed at various substrate temperatures. ( a ) Chopped photocurrent density-potential curves, ( b ) corresponding Mott–Schottky curves and ( c ) corresponding transit photocurrent spectra of the Cu 3 BiS 3 -based photocathodes sprayed at various substrate temperatures (360 °C, 380 °C, 400 °C and 420 °C). Source data are provided as a Source Data file . Full size image Figure 2c shows the transient photocurrent decay of the photocathodes based on the Cu 3 BiS 3 films sprayed at various substrate temperatures (360 °C, 380 °C, 400 °C and 420 °C). We found that the photocathode based on the Cu 3 BiS 3 film sprayed at 380 °C exhibited a smaller photocurrent spike and wider saturated photocurrent region, illustrating less charge carrier recombination and efficient photogenerated electron transfer within the electrode [28] . In summary, the photocathode based on the Cu 3 BiS 3 film sprayed at 380 °C invariably presented excellent charge-transfer kinetics, which may be attributed to the fact that the Cu 3 BiS 3 film sprayed at the 380 °C substrate temperature possessed fewer spurious phases, fewer bulk defects and higher crystallinity. As shown in Fig. S2 , electrochemical impedance spectroscopy (EIS) measurements were undertaken to further identify the charge-transfer kinetics mechanism of the Cu 3 BiS 3 -based photocathodes sprayed at various substrate temperature. The EIS measurements were carried out in phosphate buffer (pH = 6.5) under AM 1.5 G illumination biased at 0.3 V RHE with a frequency sweep from 100 kHz to 0.1 Hz. An equivalent circuit model (shown in the inset of Fig. S2 ) consisting of two serially connected resistor–capacitor blocks with a resistance ( R ) and a constant phase element was employed to fit the EIS results [42] . The fitted resistance parameters are shown in Table S1 , in which R s is mainly composed of the sheet resistance of the contact and external wire. R 1 is generally influenced by the transport of charge carriers inside the electrode, and R 2 represents the impedance at the electrode/electrolyte interface [33] , [34] , [35] , [36] , [37] , [38] , [39] , [40] . We found that the samples sprayed at 380 °C showed a significantly lower bulk resistance and lower interfacial/bulk recombination ratio of photoexcited carriers due to the compact film structure and appreciate crystalline quality of the Cu 3 BiS 3 film (380 °C), as shown in Fig. 1d . The Cu 3 BiS 3 films we studied below were all sprayed at 380 °C substrate temperature. The effects of the Cu:Bi molar ratio of the precursor solution on the crystallinity and purity of the sprayed Cu 3 BiS 3 films were also systematically investigated in this work. Figure S3 shows a comparison of the X-ray diffraction (XRD) patterns of Cu 3 BiS 3 films sprayed from precursor solutions with various Cu: Bi molar ratios. Clearly, all of the observed diffraction peaks of the Cu 3 BiS 3 film sprayed from the precursor solution with a Cu:Bi = 3:1 ratio corresponded well to the reference (JCPDS NO. 43-1479) [33] , [34] , [35] , [36] , [37] , [38] , [39] , [40] . Nevertheless, we observed obvious secondary phases and impurity phases, such as Cu 2-x S and Cu 3 Bi 3 S 7 (marked with a yellow background in Fig. S3 ), from the diffraction peaks of the Cu 3 BiS 3 films sprayed from the precursor solution with Cu:Bi ratios of 1:1, 2:1, 4:1 and 5:1. Meanwhile, the high intensity of sharp diffraction characteristic peaks of the Cu 3 BiS 3 film (with a Cu:Bi = 3:1 ratio) indicated its good crystallinity, which was preferred for high-performance water splitting device fabrication. Furthermore, the PEC performance of the Cu 3 BiS 3 -based photocathode as a function of various Cu:Bi molar ratios was also discussed. As we expected, the Cu 3 BiS 3 -based photocathode with a Cu:Bi = 3:1 ratio exhibited the highest photocurrent density and onset potential, as shown in Fig. S4a . We repeated the experiments many times and found the real trend, as shown in Fig. S4b . Relatively, the samples with an excess of Cu tended to show a higher PEC performance than Cu-deficient samples, but this trend was reversed when the molar ratio of Cu:Bi exceeded 3:1. Therefore, the stoichiometric samples possessed the highest PEC performance (including photocurrent density, onset potential and ABPE). The EIS spectra (Fig. S5 ) and the fitted resistance parameters results (Table S2 ) of these Cu 3 BiS 3 photocathodes also indicated that the stoichiometric samples exhibited the smallest values of R 1 ´ and R 2 ´ , which suggested less charge recombination inside of the electrode and better charge transfer at the electrode/electrolyte interface [42] . The EIS analyses were consistent with the results of linear sweep voltammetry (LSV) measurements (Fig. S4a ). As a result, the optimal Cu:Bi ratio of the precursor solution for the sprayed Cu 3 BiS 3 films was 3:1. On the basis of these studies, the Cu 3 BiS 3 film sprayed at a 380 °C substrate temperature and with a Cu:Bi = 3:1 molar ratio precursor solution was selected as the absorption layer for the Cu 3 BiS 3 photocathode. In this context, transmission electron microscopy (TEM) of the optimum Cu 3 BiS 3 film (Fig. S6a ) further confirmed the large Cu 3 BiS 3 crystalline size of ~1000 nm. The STEM-EDX elemental mappings of Cu, Bi and S in Fig. S6 b–d clearly showed that the elements were homogeneously distributed in the grains. In addition, the high-resolution transmission electron microscopy image of the as-prepared Cu 3 BiS 3 crystals (Fig. S6e ) indicated that the measured interplanar distance of 2.8 Å and 3.0 Å corresponds to the (131) and (102) plane of the Wittichenite Cu 3 BiS 3 (PDF No. 43-1479). The typical selected area electron diffraction pattern (Fig. S6f ) indicated that our Cu 3 BiS 3 film possessed a good crystalline quality. PEC performance of the Cu 3 BiS 3 -based photocathode As we have found in the CZTS-based photocathode, surface coverage of the CdS buffer layer is an effective way to enhance the PEC performance due to the p–n junction formed at the interface of CZTS/CdS [16] , [25] , [26] , [28] , and further deposition of the TiO 2 protective layer under CdS would enhance the PEC stability [43] . In this work, a TiO 2 /CdS overlayer and a Pt particle catalyst were also modified under the Cu 3 BiS 3 absorption layer, and the detailed deposition processes of these modification layers are given in the Supporting Information . The microscopic cross-sectional structure of the finished Pt-TiO 2 /CdS/Cu 3 BiS 3 electrode is shown in Fig. S7a , indicating that a very thin TiO 2 (~50 nm)/CdS (~80 nm) double layer was modified onto the surface of the Cu 3 BiS 3 layer (~1000 nm). The EDS mapping results (Fig. S7 b–d) clearly show the interfaces between the multilayer structure of TiO 2 /CdS/Cu 3 BiS 3 , demonstrating the compact coverage or passivation of the Cu 3 BiS 3 films by CdS and TiO 2 over layers. The PEC performances of the Pt-Cu 3 BiS 3 , Pt-CdS/Cu 3 BiS 3 and Pt-TiO 2 /CdS/Cu 3 BiS 3 photocathodes were investigated by LSV, as shown in Fig. 3a . Pt catalytic particles are necessary to provide active sites for surface reactions [43] . However, the Pt-Cu 3 BiS 3 photocathode exhibited a poor photocurrent density that was even <1 mA/cm 2 . As a buffer layer, a chemical bath deposited (CBD) CdS layer was modified onto the Cu 3 BiS 3 layer to enhance the PEC performance of the photocathodes, which was usually applied onto various absorber layers, such as CZTS and GeSe, to form heterojunctions in our previous work [25] , [43] . Accompanied by the modification of the CBD-CdS layer, the photocurrent density and onset potential of the Pt-CdS/Cu 3 BiS 3 photocathodes were substantially improved to ~2 mA/cm 2 (at 0 V RHE ) and ~0.75 V RHE , respectively. The enhancement of the PEC performance was attributed to the heterojunction that was formed at the interface of CdS/Cu 3 BiS 3 , which can efficiently promote the separation of charge carriers and reduce surface recombination [25] , [43] . Fig. 3: PEC performance of the Cu 3 BiS 3 -based photocathodes. ( a ) Chopped photocurrent density-potential curves of the Pt-Cu 3 BiS 3 , Pt-CdS/Cu 3 BiS 3 and Pt-TiO 2 /CdS/Cu 3 BiS 3 photocathodes. ( b ) ABPE curves, ( c ) IPCE spectra and ( d ) photocurrent density-time curves of the Pt-CdS/Cu 3 BiS 3 and Pt-TiO 2 /CdS/Cu 3 BiS 3 photocathodes. ( e ) Hydrogen and oxygen evolution amounts of the Pt-TiO 2 /CdS/Cu 3 BiS 3 photocathode with various illumination times and ( f ) photograph of the Pt-TiO 2 /CdS/Cu 3 BiS 3 photocathode under working conditions. All measurements were carried out in a 0.2 mol/dm 3 Na 2 HPO 4 /NaH 2 PO 4 solution (pH = 6.5) under solar simulated AM 1.5 G light irradiation. Source data are provided as a Source Data file . Full size image Nevertheless, the photocurrent density of the Pt-CdS/Cu 3 BiS 3 photocathode was less than half of the initial value after the 3 h stability test, as shown in Fig. 3d , due to the oxidative self-photocorrosion of the CdS layer [25] . Consequently, a protective TiO 2 layer deposited by atomic layer deposition (ALD) was modified onto the surface of the CdS layer to achieve relatively stable photocathodes in this work, which is a conventional strategy to enhance the stability of previously reported photocathodes such as CZTS [44] , Cu 2 BaSn(S, Se) 4 [45] , Cu(In,Ga)Se 2 [13] , GeSe [43] , Sb 2 Se 3 [41] and Cu 2 O [31] . To our surprise, as shown in Fig. 3a and d, not only was the stability of the photocathodes significantly improved to over 10 h but also the photocurrent density dramatically increased from ~2 mA/cm 2 to ~7 mA/cm 2 (at 0 V RHE ), and the onset potential increased to above ~0.9 V RHE with the modification of the TiO 2 layer. Meanwhile, there were no obvious corrosive metamorphisms at the surface of the finished photocathodes by comparing the cross-sectional SEM images before and after the 10 h stability test (Fig. S8 ), further confirming the great protective effect of the pinhole-free ALD-TiO 2 layer. It should be emphasized that such a relatively high onset potential of ~0.9 V RHE provides the conditions for the realization of efficient unbiased water splitting cells in contact with appropriate photoanodes such as BiVO 4 and Fe 2 O 3 [29] , [30] . Moreover, the finished photocathode achieved the highest ABPE of 1.7% at 0.4 V RHE , which was more than four times that of the Pt-CdS/Cu 3 BiS 3 photocathode, as shown in Fig. 3b . The protective effect of the TiO 2 layer can be referenced to previous related works [13] , [31] , [41] , [43] , [45] , and the underlying mechanism of the increased PEC performance of the inserted TiO 2 layer was further understood through a series of PEC characterizations and band schema. 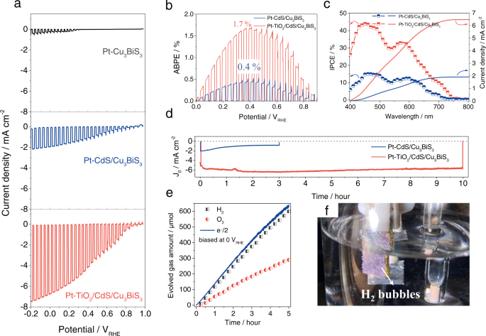Fig. 3: PEC performance of the Cu3BiS3-based photocathodes. (a) Chopped photocurrent density-potential curves of the Pt-Cu3BiS3, Pt-CdS/Cu3BiS3and Pt-TiO2/CdS/Cu3BiS3photocathodes. (b) ABPE curves, (c) IPCE spectra and (d) photocurrent density-time curves of the Pt-CdS/Cu3BiS3and Pt-TiO2/CdS/Cu3BiS3photocathodes. (e) Hydrogen and oxygen evolution amounts of the Pt-TiO2/CdS/Cu3BiS3photocathode with various illumination times and (f) photograph of the Pt-TiO2/CdS/Cu3BiS3photocathode under working conditions. All measurements were carried out in a 0.2 mol/dm3Na2HPO4/NaH2PO4solution (pH = 6.5) under solar simulated AM 1.5 G light irradiation. Source data are provided as aSource Data file. Figure 3c shows the spectra of the incident photocurrent conversion efficiency (IPCE) undertaken at 0 V RHE and the corresponding integrated photocurrent density of the Pt-CdS/Cu 3 BiS 3 and Pt-TiO 2 /CdS/Cu 3 BiS 3 photocathodes. Accompanied by the importation of the TiO 2 layer, the increase in the IPCE in the low wavelength range was more obvious than that in the relatively long wavelength range (the IPCE value increased from 15 to 44% at 450 nm), indicating that the inserted TiO 2 layer greatly enhanced the light harvesting and conversion efficiency in the low wavelength range of the finished photocathode. It was observed that the efficiency dropped suddenly in the wavelength range of 490–540 nm with a long absorption tail after 590 nm for the finished photocathodes, suggesting that the interfacial recombination of photoexcited carriers in the Pt-TiO 2 /CdS/Cu 3 BiS 3 photocathode was still obvious. Whether the TiO 2 layer was introduced or not, the integrated photocurrent density practically matched the photocurrent density measured by LSV, demonstrating the uniformity of LSV measurements and IPCE results. In addition, the reflection characterizations (Fig. S9 ) of our Cu 3 BiS 3 -based photocathodes with and without TiO 2 layer also demonstrated that the TiO 2 layer can be used as an antireflection layer to enhance the light absorption for the Cu 3 BiS 3 -based photocathodes. Furthermore, intensity-modulated photovoltage spectroscopy (Fig. S10 ) and intensity-modulated photocurrent spectroscopy (Fig. S11 ) of the three electrodes (Pt-Cu 3 BiS 3 , Pt-CdS/Cu 3 BiS 3 , and Pt-TiO 2 /CdS/Cu 3 BiS 3 ) were performed to understand the surface/interfacial recombination or transfer of photogenerated carriers in the electrodes. Through the calculation (the detailed computational procedures are given in the Supporting Information ), the Pt-TiO 2 /CdS/Cu 3 BiS 3 photocathode exhibited a higher carrier lifetime ( τ n ) and a lower charge transfer time ( τ d ) than those of the Pt-Cu 3 BiS 3 and Pt-CdS/Cu 3 BiS 3 photocathodes, which indicated that the transfer efficiency of the photoexcited carriers was enhanced and the interfacial recombination rate was decreased with the importation of the TiO 2 /CdS overlayer [46] . The band diagram of the TiO 2 /CdS/Cu 3 BiS 3 electrode was further investigated, as shown in Fig. S12 . There was a conspicuous cliff-like conduction band offset (0.7 eV) at the interface of CdS/Cu 3 BiS 3 , which would result in a recombination center at the interface and be unbeneficial for the transfer of the photogenerated electrons [33] . This is also one of the reasons why the previously reported Cu 3 BiS 3 -based photovoltaic devices presented a poor conversion efficiency buffered with a CdS layer [35] , [37] . Accompanied by the inserted ALD-TiO 2 layer, the photogenerated electrons and holes can be separated more effectively due to the relatively low valence band position of TiO 2 . Moreover, the photogenerated electrons can also be selectively transferred through the TiO 2 layer directly into the electrolyte and participate in the hydrogen evolution reaction [24] . Based on the above discussion, these factors all led to a higher PEC performance for the Pt-TiO 2 /CdS/Cu 3 BiS 3 photocathode than the photocathode modified with a single CdS layer. Figure 3e shows the H 2 and O 2 production amounts of the finished photocathode biased at 0 V RHE with various illumination times. H 2 gas was produced with a constant rate of 141 µmol cm −2 h −1 , indicating the highly stable overall solar water splitting properties of the Pt-TiO 2 /CdS/Cu 3 BiS 3 photocathode. Notably, the H 2 and O 2 production amounts of the finished photocathode biased at more positive potentials (such as 0.3 V RHE and 0.6 V RHE ) were also determined, and as shown in Fig. S13 , H 2 gas can be produced steadily with constant rates of 95.7 µmol cm −2 h −1 and 35.2 µmol cm −2 h −1 , respectively, when the finished photocathode was biased at 0.3 V RHE and 0.6 V RHE under simulated solar irradiation, which further identified the authenticity of such a high onset potential (~0.9 V RHE ) of the Pt-TiO 2 /CdS/Cu 3 BiS 3 photocathode. Meanwhile, according to our calculation, the faradaic efficiency of this Pt-TiO 2 /CdS/Cu 3 BiS 3 photocathode biased at any potential (0 V RHE , 0.3 V RHE and 0.6 V RHE ) were all close to 90% (Fig. S14 ). Figure 3f is a photograph of the Pt-TiO 2 /CdS/Cu 3 BiS 3 photocathode under working conditions. The thickness of the CdS buffer was found to significantly influence the PEC properties of the Cu 3 BiS 3 -based photocathode, and the statistical results are shown in Fig. S15 . It was found that the optimum thickness of the CdS buffer was ~80 nm (i.e., 15 min CBD). A thinner CdS buffer (i.e., <80 nm) may not efficiently passivate the surface of Cu 3 BiS 3, while a thicker CdS buffer (higher than 80 nm) would increase the resistance and absorb solar light without passing through the Cu 3 BiS 3 photoabsorber (Fig. S16 ). In addition, a CdS layer that is too thick may increase the photoexcited carrier recombination efficiency, as shown in the transit photocurrent spectra (Fig. S17 ). On the basis of these studies, the optimum deposition time of the CBD-CdS layer was determined to be 15 min in this work, and the thickness of the CBD-CdS layer deposited for 15 min can reach ~80 nm (Fig. S7 ) Scalable Cu 3 BiS 3 -BiVO 4 tandem cell for unbiased solar water splitting It should be noted here that the Cu 3 BiS 3 -based photocathode presented a very promising solar water splitting photovoltage >0.9 V RHE , and such a high onset potential is very important and suitable to assemble efficient tandem of photocathode-photoanode cells for standalone devices. In this work, we prepared a tandem cell of Cu 3 BiS 3 -BiVO 4 . 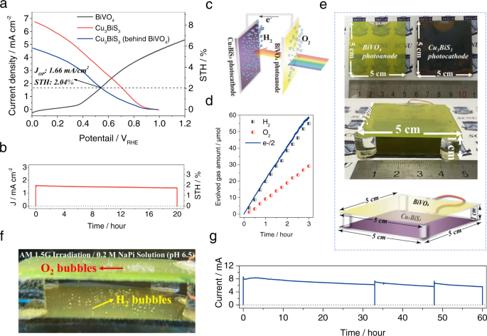Fig. 4: PEC performance of the scalable Cu3BiS3-BiVO4tandem device. (a) J–V curves of the Cu3BiS3photocathode, BiVO4photoanode and Cu3BiS3photocathode behind the BiVO4photoanode. (Jop: the operation point photocurrent density, STH: solar to hydrogen efficiency). (b) Photocurrent density-time curve, (c) working diagram and (d) hydrogen and oxygen evolution amount-time curves of the Cu3BiS3-BiVO4tandem device. (e) Photographs of the 5 × 5 cm2Cu3BiS3photocathode, 5 × 5 cm2BiVO4photoanode and large area (5 × 5 cm2) Cu3BiS3-BiVO4tandem device and diagram of the large area (5 × 5 cm2) Cu3BiS3-BiVO4tandem device. (f) Working photograph of the large area (5 × 5 cm2) Cu3BiS3-BiVO4tandem device under solar simulated AM 1.5 G irradiation. (g) Photocurrent density-time curve of the large area (5 × 5 cm2) Cu3BiS3-BiVO4tandem device. All measurements were carried out in a 0.2 mol/dm3Na2HPO4/NaH2PO4solution (pH = 6.5) under solar simulated AM 1.5 G irradiation. Source data are provided as aSource Data file. 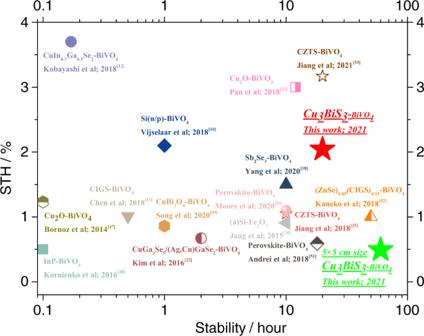Fig. 5: Benchmarks for previously reported photocathode-photoanode tandem cells. Efficiency and stability benchmarks of the previously reported photocathode-photoanode tandem cells for standalone water splitting. The statistical PEC performance parameters are shown in Table1. Figure 4a shows the current-potential curves obtained from a Cu 3 BiS 3 -based photocathode and a BiVO 4 photoanode; thus, a two-electrode tandem PEC cell was assembled by placing a BiVO 4 /FTO photoanode (0.73 cm 2 ) in front of a Pt-TiO 2 /CdS/Cu 3 BiS 3 photocathode (0.45 cm 2 ) followed by exposure to simulated AM 1.5 G solar radiation, as shown in Fig. S18 . The details of the synthesis of the efficient BiVO 4 photoanode were illustrated in our previous paper [29] . There was an obvious duplication between the J–V curves of the Cu 3 BiS 3 photocathode and BiVO 4 photoanode under a photovoltage from 0.35 V RHE to 0.9 V RHE , and the crossing point and operation point were observed at 1.66 mA/cm 2 ( J op ) and 0.54 V RHE , respectively. We showed the video of the Cu 3 BiS 3 -BiVO 4 tandem cell under working with simulated sunlight irradiation (Movie S1 ) in Supporting Information , many H 2 /O 2 bubbles were evolved from the tandem cell for the overall solar water splitting reaction. Meanwhile, the IPCE spectra (Fig. S19 ) measured under the operating bias (0.54 V RHE ) for both electrodes show complimentary spectral responses. The energy band diagrams of the Cu 3 BiS 3 -BiVO 4 tandem cell (Fig. S20 ) show the photogenerated carrier transfer path and solar hydrogen evolution reaction process. Based on the STH efficiency calculation equation: 
    η_STH=(J_op× 1.23)/P
 (1) where P is the power of the illuminating light, the STH of this Cu 3 BiS 3 -BiVO 4 tandem cell achieved a remarkable efficiency of 2.04%. This 2.04% STH efficiency is the first reported and recorded unbiased STH efficiency for Cu 3 BiS 3 -BiVO 4 tandem cells, which is very close to the record STH efficiency from Cu 2 O-BiVO 4 tandem cells reported by the Gratzel group (Table 1 ) [31] . Fig. 4: PEC performance of the scalable Cu 3 BiS 3 -BiVO 4 tandem device. ( a ) J–V curves of the Cu 3 BiS 3 photocathode, BiVO 4 photoanode and Cu 3 BiS 3 photocathode behind the BiVO 4 photoanode. (Jop: the operation point photocurrent density, STH: solar to hydrogen efficiency). ( b ) Photocurrent density-time curve, ( c ) working diagram and ( d ) hydrogen and oxygen evolution amount-time curves of the Cu 3 BiS 3 -BiVO 4 tandem device. ( e ) Photographs of the 5 × 5 cm 2 Cu 3 BiS 3 photocathode, 5 × 5 cm 2 BiVO 4 photoanode and large area (5 × 5 cm 2 ) Cu 3 BiS 3 -BiVO 4 tandem device and diagram of the large area (5 × 5 cm 2 ) Cu 3 BiS 3 -BiVO 4 tandem device. ( f ) Working photograph of the large area (5 × 5 cm 2 ) Cu 3 BiS 3 -BiVO 4 tandem device under solar simulated AM 1.5 G irradiation. ( g ) Photocurrent density-time curve of the large area (5 × 5 cm 2 ) Cu 3 BiS 3 -BiVO 4 tandem device. All measurements were carried out in a 0.2 mol/dm 3 Na 2 HPO 4 /NaH 2 PO 4 solution (pH = 6.5) under solar simulated AM 1.5 G irradiation. Source data are provided as a Source Data file . Full size image Table 1 PEC performance of previously reported typical photocathodes and their tandem cell modules. Full size table Stability is another important issue to evaluate the real application potential, and we characterized the long-term photocurrent stability of this Cu 3 BiS 3 -BiVO 4 tandem cell over 20 h of irradiation (AM 1.5 G). The data shown in Fig. 4b demonstrate that the tandem cell possessed a very high long-term stability, and the photocurrent after 20 h of irradiation maintained ~90% of its initial value. The working diagram of this tandem cell is shown in Fig. 4c . In addition, Fig. 4d shows that the Cu 3 BiS 3 -BiVO 4 tandem cell possessed stable H 2 gas evolution with a constant ratio of 18 µmol/h. The appreciable efficiency and high stability of the Cu 3 BiS 3 photocathode and the Cu 3 BiS 3 -BiVO 4 tandem cell are very suitable for practical utilizations. However, the device size is another key point. Fortunately, large Cu 3 BiS 3 and BiVO 4 photoelectrodes are not difficult to obtain. We prepared 5 × 5 cm 2 Cu 3 BiS 3 and BiVO 4 and assembled them into a tandem device in this work, and their photos and the model diagram are shown in Fig. 4e . The 5 × 5 cm 2 size Cu 3 BiS 3 photocathode not only presented an appreciable photocurrent of about 90 mA under 0 V RHE (active area: 21 cm 2 ) but also possessed an excellent working stability (Fig. S21 ). Significant number of H 2 bubbles were observed to be continuously produced from the surface of Cu 3 BiS 3 photocathode under simulated sunlight irradiation (Movie S2 , Fig. S22 ). It should be noted here that 5 × 5 cm 2 is the largest size we can currently prepare due to the limit of our apparatus, and much larger sizes, such as 10 × 10 cm 2 or 20 × 20 cm 2 , should be able to be prepared when we update our apparatus. Figure 4f and Movie S3 show a photograph and a video of this 5 × 5 cm 2 Cu 3 BiS 3 -BiVO 4 tandem device under simulated AM 1.5 G solar light illumination, respectively. Many H 2 and O 2 bubbles can be observed on the surface of the Cu 3 BiS 3 photocathode and BiVO 4 photocathode, respectively. As shown in Fig. 4g , the photocurrent of this 5 × 5 cm 2 Cu 3 BiS 3 -BiVO 4 tandem device did not obviously decrease even over the 60 h stability test, indicating that the long-term operation of the large Cu 3 BiS 3 -BiVO 4 tandem device is promising. Although the photocurrent of the Cu 3 BiS 3 -based photocathodes in this work still has much room for improvement, the photovoltage and stability of the Cu 3 BiS 3 photocathode presented here are very close to the record of the Cu 2 O photocathode [31] but already higher than those of various typical photocathodes, such as CZTS [25] , CIGS [12] , Sb 2 Se 3 [18] , Si [10] and so on (Table 1 ). We can expect large potential for the improvement in the PEC properties of Cu 3 BiS 3 -based photocathodes. Compared with Cu 2 O, we found that the Cu 3 BiS 3 film is relatively stable in neutral buffer solutions and that the stable Cu 3 BiS 3 film is much easier to obtain than Cu 2 O [31] . We believe that the Cu 3 BiS 3 -based photocathode will attract much attention and be significantly improved in the near future. The over 2% STH efficiency of the Cu 3 BiS 3 -BiVO 4 tandem devices and over 20 h of stability presented indicate great potential for solar water splitting. In comparison with the previously reported typical tandem cell (Fig. 5 ), it was found that the STH efficiency of our Cu 3 BiS 3 -BiVO 4 tandem cell was competitive among them. Nevertheless, it should be noted that the research of the Cu 3 BiS 3 photoelectrode is almost at the starting point now, and the presented appreciable STH efficiency (2.04%) and stability (20 h and 60 h) indicate great potential for Cu 3 BiS 3 photoelectrodes. We believe that the PEC efficiency/stability of the Cu 3 BiS 3 photoelectrode and Cu 3 BiS 3 -BiVO 4 tandem cell will be significantly improved and even higher than those of other famous CIGS-, Cu 2 O- and CZTS-based photoelectrodes in the near future. This work provides a promising starting point for the development of Cu 3 BiS 3 -based photoelectrodes, and we believe that one milestone after another will be achieved in the future. Fig. 5: Benchmarks for previously reported photocathode-photoanode tandem cells. Efficiency and stability benchmarks of the previously reported photocathode-photoanode tandem cells for standalone water splitting. The statistical PEC performance parameters are shown in Table 1 . Full size image In this work, the Cu 3 BiS 3 -based photocathode exhibited excitation at a set potential over 0.9 V RHE and an excellent PEC current density of ~7 mA/cm 2 under 0 V RHE with 10 h long-term high stability in neutral water solutions. Further fabricated Cu 3 BiS 3 -BiVO 4 photocathode-to-photoanode tandem cells presented a good unbiased STH conversion efficiency as high as 2.04%. However, such tandem devices also presented superior high stability over 20 h. Finally, a 5 × 5 cm 2 large Cu 3 BiS 3 -BiVO 4 tandem device module was fabricated for scalable overall solar water splitting device applications, and the stable photocurrent of this larger module over 60 h of operation under sustained solar light irradiation was detected. The appreciable PEC properties, such as the high onset potential, good photocurrent, over 60 h of high stability, ideal STH efficiency (2.04%) and scalable device module (5 × 5 cm 2 ) for the Cu 3 BiS 3 -based photocathode that were presented in this work, all indicate its remarkable application value and great potential for solar water splitting. Preparation of the Cu 3 BiS 3 films The Cu 3 BiS 3 films (with a Cu/3:Bi = 1 mole ratio) were prepared by spray pyrolysis method. The sprayed precursor solution was mixed by 15 mL CuCl-Tu (excess) DMSO solution and 15 mL BiCl 3 - Tu (excess) DMSO solution. Specifically, the Cu-Tu stock solution was formed by 2.97 g CuCl (2 M) and excess thiourea (Tu) both dissolved in 15 mL DMSO, and the Bi-Tu stock solution was formed by 3.15 g BiCl 3 (0.666 M) and excess thiourea (Tu) both dissolved in 15 mL DMSO. Then, the two stock solutions were both separately stirred until clear and transparent before their mix. Furthermore, the mixing CuCl (1 M), BiCl 3 (0.333 M) and excess Tu precursor solution was also stirred for 5 h, ultimately obtaining a yellow clear sprayed solution for Cu 3 BiS 3 films preparation. The precursor solution was subsequently sprayed onto a cleaned Mo-coated soda-lime glass substrate preheated to 380 °C for about 3 min. Surface mdification with TiO 2 /CdS overlayer First, a CdS layer was deposited under the Cu 3 BiS 3 layer by the chemical bath deposition method (CBD). The prepared Cu 3 BiS 3 layer was dipped into an aqueous solution containing 12.5 mM CdSO 4 , 0.22 mM SC(NH 2 ) 2 , and 11 M NH 4 OH at 60 °C for 15 min. Furthermore, a TiO 2 layer was deposited under the CdS/Cu 3 BiS 3 double layer by ALD method. The TiO 2 layer was grown by using titanium tetrakis (dimethylamide) as titanium source and H 2 O as oxygen source. Based on our empirical value, the growth rate was estimated to be about 0.054 nm per cycle and the TiO 2 film was grown for 926 cycles at 120 °C, and the corresponding thicknesses of the TiO 2 layer was 50 nm, ultimately obtaining a TiO 2 /CdS/Cu 3 BiS 3 electrode. Deposition of Pt particles The Pt particles deposition was performed by using a three-electrode system consisting of TiO 2 /CdS/Cu 3 BiS 3 as a working electrode, a Pt wire as a counter electrode, and Ag/AgCl as a reference electrode. These electrodes were put in 0.1 M Na 2 SO 4 solution containing 1 mM H 2 PtCl 6 , and the deposition was performed with a constant potential of −0.1 V Ag/AgCl by using CHI660E electrochemical measurement unit. During the deposition process, the working electrode was illuminated by simulated AM 1.5 G solar irradiation. Preparation of the BiVO 4 photoanodes The BiVO 4 films were also prepared by spray pyrolysis method. The sprayed solution was prepared by dissolving Bi(NO 3 ) 3 ·5H 2 O in acetic acid and VO(AcAc) 2 in absolute ethanol. The Bi stock solution was then added into the V stock solution, and the mixture was diluted to 4 mM with excess ethanol. The mixed precursor solution was immediately sprayed onto a cleaned FTO-coated glass substrate preheated to 450 °C, and the spray nozzle was placed 25 cm above the heating plate. The sprayed solution was driven by an over pressure of 0.5 bar of N 2 gas. Photoelectrochemical measurements An online gas chromatography system (Shimadazu GC-2014 gas analyzer equipped with a MS-5A column and a thermal conductivity detector) was used to detect H 2 and O 2 during the PEC water splitting. PEC H 2 generation from photocathodes was examined in a pH 6.5 phosphate buffer solution (0.2 M Na 2 HPO 4 /NaH 2 PO 4 ) by using the above-mentioned solar simulator as a light source. The PEC cell was covered by a water jacket to maintain the temperature at 293 K. The two-electrode setup composed of the Pt-TiO 2 /CdS/Cu 3 BiS 3 photocathode and a BiVO 4 photoanode in series connection was also employed to examine water splitting under the bias-free condition. Furthermore, the phosphate buffer solution was updated per 20 h stability test to keep the concentration (0.2 M) and pH (6.5) unchanged. The intensity of simulated sunlight was also calibrated per 20 h stability test. Potentials referred to the Ag/AgCl electrode were converted to reversible hydrogen electrode using the Nernst equation: 
    V_RHE=V_Ag/AgCl+0.059× pH+0.199
 (2) ABPE was determined from the current density−potential response of the photocathodes by using the following equation: 
    ABPE  ( % )=J× V× 100/P
 (3) Where J is the photocurrent density (mA/cm 2 ), V is the applied potential (V RHE ), and P is the intensity of simulated sunlight (100 mW/cm 2 ). Structural characterization Crystalline structures of the films were determined by XRD, Raman spectroscopy and TEM using a Rigaku Mini Flex X-ray diffractometer, a Jasco NRC 3100 laser Raman spectrophotometer and JEOL JEM-2100HR microscope respectively. Surface and cross section morphology were observed by scanning electron microscope (SEM) using Hitachi S-4800 micros.